Three-dimensional analysis of ribonucleoprotein complexes in influenza A virus The influenza A virus genome consists of eight single-stranded negative-sense RNA (vRNA) segments. Although genome segmentation provides advantages such as genetic reassortment, which contributes to the emergence of novel strains with pandemic potential, it complicates the genome packaging of progeny virions. Here we elucidate, using electron tomography, the three-dimensional structure of ribonucleoprotein complexes (RNPs) within progeny virions. Each virion is packed with eight well-organized RNPs that possess rod-like structures of different lengths. Multiple interactions are found among the RNPs. The position of the eight RNPs is not consistent among virions, but a pattern suggests the existence of a specific mechanism for assembly of these RNPs. Analyses of budding progeny virions suggest two independent roles for the viral spike proteins: RNP association on the plasma membrane and the subsequent formation of the virion shell. Our data provide further insights into the mechanisms responsible for segmented-genome packaging into virions. Influenza A viruses are enveloped, with an elliptical or filamentous shape, ranging from 80 to 120 nm in diameter [1] . The virions are covered with viral spike proteins, hemagglutinin (HA), neuraminidase (NA) and an ion channel protein (M2). The eight negative-sense RNA (vRNA) segments of the genome range in size from 890 to 2,341 bases [1] . Each vRNA segment associates with a nucleoprotein scaffold and an RNA-dependent RNA polymerase complex to form a rod-like ribonucleoprotein (RNP) of approximately 13 nm in diameter [1] . The rod-like RNPs vary in length from 30 to 110 nm, which correlates with the length of each vRNA segment [2] . The structures of purified RNPs from virions [2] , [3] , [4] as well as those of recombinant RNPs generated in vitro from NP, RNA polymerase complex and the short vRNA-like genome [5] , [6] , [7] , have been characterized by use of electron microscopy (EM). However, information about the structures of the RNPs inside virions is limited. Previously, we used conventional ultra-thin section EM to show that eight RNPs of different lengths are arranged in a specific pattern, with seven RNPs surrounding a central one in each budding virion [8] . However, three-dimensional (3-D) structures of RNPs inside the virions, as well as knowledge of the detailed spatial organization inside the virions, are still lacking. Here, to construct and investigate the 3-D structure of the RNPs within progeny virions, we used scanning transmission EM (STEM) tomography, which is a new technique in life sciences and provides a better contrast and signal-to-noise ratio than that of conventional bright-field transmission electron tomography [9] , [10] . Although STEM tomography suffers from an artifact, namely the missing wedge effect, similar to conventional electron tomography [9] , the dual-axis STEM tomography we used in this study substantially reduces the missing wedge effect [11] , resulting in fewer artifacts in the reconstructed images. 3-D structure of the eight RNPs within budding virions By using STEM, we examined thin sections (approximately 200 nm thick) of virus-infected cells and captured areas of interest for 3-D reconstruction ( Supplementary Fig. S1 ). A series of tomograms of progeny virions shows that all virions examined contained rod-like RNPs of approximately 12 nm in diameter ( Fig. 1 ; Supplementary Movie 1 ). Transversely sectioned progeny virions clearly shows the eight RNPs arranged in a distinct pattern, in which a central RNP is surrounded by seven RNPs ( Supplementary Movie 1 ), as demonstrated previously by using conventional ultrathin-section EM [8] , [12] . The consecutive 0.5-nm thick tomograms through a whole virion at 5.0 nm intervals, which were computationally generated from a 3-D reconstructed virion, demonstrate that all eight RNPs are associated with the interior of the budding front of the virion and that the eight RNPs differ in length, with three long RNPs of similar lengths ( Fig. 1a ), consistent with the lengths of the eight vRNA segments [1] . The eight RNPs appear well organized; however, serial images through the z axis of the virion depict a progressive shift of each RNP cross-section in a random manner ( Fig. 1a ; Supplementary Movie 2 ), indicating that they are not arranged strictly with sevenfold symmetry. These results depict the 3-D model of RNPs within progeny virions; the eight RNPs within the virion are well organized but asymmetrically arranged, and respective RNPs are not straight rods, but are flexible serpentine-curved structures, consistent with a study showing that nucleoprotein oligomerization is mediated by a flexible tail loop [13] . The eight RNPs are packed densely within the lipid envelope that is covered with glycoprotein spikes protruding outward from the surface ( Fig. 1b ; Supplementary Movies 3 and 4 ). Some peripheral RNPs appear to be associated with the lipid envelope as reported previously [14] ( Fig. 1a ), although the biological significance of this association is unclear. 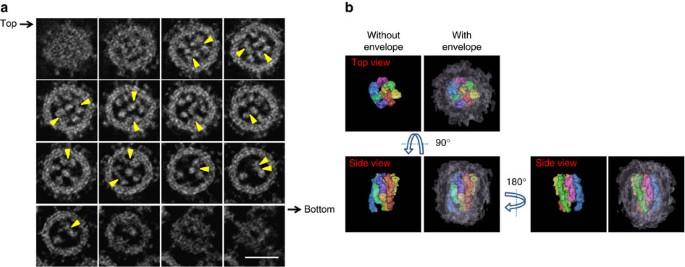Figure 1: Dual-axis STEM tomography of a progeny influenza A virion. (a) Consecutive transverse sections of a progeny virion (0.5 nm thick at 5.0-nm intervals) from its top to bottom. The RNPs, approximately 12 nm in diameter, are present within the viral envelope. Representative associations between the RNPs are shown as examples (arrowheads). Scale bar, 50 nm. (b) A 3-D model of the eight RNPs within a virion. Each RNP and the viral envelope are represented by a different colour. Figure 1: Dual-axis STEM tomography of a progeny influenza A virion. ( a ) Consecutive transverse sections of a progeny virion (0.5 nm thick at 5.0-nm intervals) from its top to bottom. The RNPs, approximately 12 nm in diameter, are present within the viral envelope. Representative associations between the RNPs are shown as examples (arrowheads). Scale bar, 50 nm. ( b ) A 3-D model of the eight RNPs within a virion. Each RNP and the viral envelope are represented by a different colour. Full size image Interactions among the eight RNPs inside the virions Because interactions among RNPs are required to form and maintain the specific arrangement of the eight RNPs, we then looked for physical associations among the eight RNPs. Tomograms (0.5 nm thick), in which overlapping features caused by two-dimensional projection in 3-D objects are practically negligible, revealed frequent direct contacts between the RNPs ( Fig. 1a , arrowheads). These contacts were observed between peripheral RNPs as well as between central and peripheral RNPs throughout the virion. We also found linkages between the RNPs via short string-like structures ( Fig. 2 , Supplementary Fig. S2 ; Supplementary Movie 2 ). These short string-like structures were approximately 2 nm in diameter and, at most, 10 nm in length, such that they linked only adjacent RNPs ( Fig. 2 ; Supplementary Fig. S2 , arrowheads). Importantly, these string-like structures were always found between the RNPs; they were never observed dissociated from the RNPs within virions. These findings suggest that although a specific interaction pattern was not found, there are physical multi-interactions among the eight RNPs, possibly involved in their selective genome packaging [15] , [16] , [17] . Although the nature of these short string-like structures remains unknown, their existence as RNP linkers is potentially important, because their fibril shape resembles that of RNA [18] . It is known that RNAs are recognized as structures as well as nucleotide sequences [19] , [20] , which could sort the eight vRNA segments via specific RNA–RNA interactions with the segment-specific packaging signals that exist on the eight vRNA segments [15] , [16] , [17] . 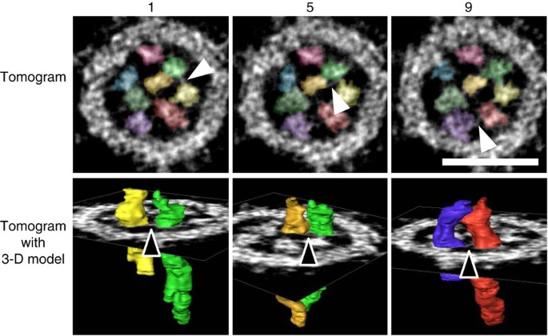Figure 2: Linkages among the eight RNPs in a virion. Short string-like structures of approximately 2 nm in diameter can be seen between the RNPs (arrowheads). Tomograms, 0.5-nm thick, are shown in the upper row. The 3-D models of two RNPs connected by a string-like structure are shown in the lower row. Virtual slice numbers (1, 5 and 9) of 0.5-nm thick tomograms are given above the tomograms. The colour scheme of the RNPs is the same as that shown inFigure 1b. Scale bar, 50 nm. Figure 2: Linkages among the eight RNPs in a virion. Short string-like structures of approximately 2 nm in diameter can be seen between the RNPs (arrowheads). Tomograms, 0.5-nm thick, are shown in the upper row. The 3-D models of two RNPs connected by a string-like structure are shown in the lower row. Virtual slice numbers (1, 5 and 9) of 0.5-nm thick tomograms are given above the tomograms. The colour scheme of the RNPs is the same as that shown in Figure 1b . Scale bar, 50 nm. Full size image Organization of the eight RNPs in multi-segment complexes The major advantage of electron tomography over conventional ultrathin-section EM is the availability of 3-D spatial information. To determine whether the structural arrangement of the eight RNPs is common among different progeny virions, we generated 3-D models of the multi-segment complex from 30 progeny virions, which were randomly picked. All virions contained eight RNPs arranged in the distinct pattern, suggesting that the eight RNPs are commonly packaged into progeny virions. In most virions examined, the bottom ends of the three long RNPs were not included in the 200-nm thick sections and were thus truncated in the 3-D models; the other five RNPs were included in their entirety within the sections and successfully reconstructed. 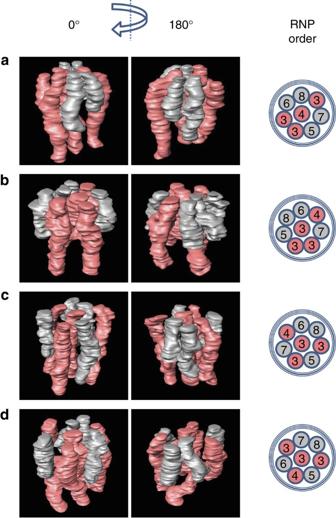Figure 3: 3-D models of the eight RNPs in different virions. (a?d) Four examples of 3-D models of the multi-segment complex are shown. The schemes illustrated in the right column show the order of the eight RNPs, which are numbered from 3 to 8 in descending order of length (that is, 3, 3, 3, 4, 5, 6, 7 and 8). For clarity, the four longer RNPs (that is, numbers 3, 3, 3 and 4) are coloured red and the four shorter RNPs (that is, numbers 5, 6, 7 and 8) are coloured grey. Figure 3 shows how the multi-segment complex was slightly different among virions, although they all retained the 7+1 arrangement. In some multi-segment complexes, the RNPs appeared to unite at the top of the virion ( Fig. 3a,b ), whereas, in other instances, each RNP was oriented almost perpendicular to the top of the virion and seemed to be isolated from its neighbour ( Fig. 3c,d ), suggesting that the 3-D architecture of the multi-segment complex is heterogeneous among virions. Given that the nucleoprotein oligomer shows inherent flexibility [13] , it is plausible that the architecture of the multi-segment complex would not be rigid within live virions. Figure 3: 3-D models of the eight RNPs in different virions. ( a?d ) Four examples of 3-D models of the multi-segment complex are shown. The schemes illustrated in the right column show the order of the eight RNPs, which are numbered from 3 to 8 in descending order of length (that is, 3, 3, 3, 4, 5, 6, 7 and 8). For clarity, the four longer RNPs (that is, numbers 3, 3, 3 and 4) are coloured red and the four shorter RNPs (that is, numbers 5, 6, 7 and 8) are coloured grey. Full size image To further characterize the architecture of the multi-segment complex within progeny virions, we examined the order of configuration of the eight RNPs based on their different lengths. The eight RNPs were numbered in descending order of length. Because the ends of the three long RNPs were often excluded from the 200-nm thick sections, all the three long RNPs were assigned the number 3, and the other five RNPs of different lengths were assigned different numbers (that is, the eight RNPs were assigned the numbers 3, 3, 3, 4, 5, 6, 7 and 8, where 3 is assigned to the longest RNPs and 8 to the shortest). The differences in length between number 4 and 5, 5 and 6, 6 and 7, and 7 and 8 segments were 9.9±2.1, 4.1±1.9, 3.7±1.9 and 6.9±2.4 nm, respectively ( Supplementary Fig. S3a ). On the basis of these measurements, the differences in length between the respective RNP pairs were similar among the 30 virions examined here, suggesting that the assignment of the eight RNPs is reliable. Furthermore, we found that the differences in length between segment numbers 4 and 8, 5 and 8, 6 and 8, and 7 and 8 were statistically significant ( Supplementary Fig. S3b ), indicating that the shorter five RNPs (that is, segment numbers 4, 5, 6, 7 and 8) are different in length. Together with the observation that all virions examined here contain three long RNPs, these data strongly suggest that budding virions contain eight different RNPs. The order of the eight RNPs in the multi-segment complex was different among all 30 virions examined here ( Fig. 3 ; Supplementary Fig. S4 ). However, the central RNP in the specific arrangement was consistently long (a number 3 or 4), with a probability of <0.001% (see Methods), suggesting some structural role for the central RNP. Furthermore, the remaining three long RNPs did not sequentially line up among the seven peripheral RNPs ( Supplementary Figs S4 and S5b ). Although the three long RNPs could theoretically line up sequentially in the seven peripheral positions ( Supplementary Fig. S5a ) 20% of the time, such an arrangement was not found in the 30 virions we examined here ( Fig. 3 ; Supplementary Fig. S4 ). This probability is <0.124% (see Methods), suggesting that these long RNPs have some structural roles or constraints. Together, our results demonstrate that the positions of the eight RNPs within virions have a characteristic pattern. Our findings also imply that the interactions among the eight RNPs are limited, and it is unlikely for every RNP to interact with all of its neighbouring RNPs to a level that would completely define its position in virions. The central RNP may not associate specifically with all of the peripheral RNPs, and every peripheral RNP may not have a specific interaction with neighbouring RNPs, otherwise, the order of the eight RNPs should be identical in all virions. The mechanisms whereby such limited interactions selectively arrange the eight different vRNA segments remain obscure. Tomographic analyses of virions during budding Finally, to investigate the packaging process of the eight RNPs into progeny virions, we used immuno EM and STEM tomography to examine virions formed during budding from the surfaces of infected cells (designated previrions). Immuno EM with anti-NP, HA or M2 antibodies demonstrated that for virions at the initial to middle phase of budding, viral spike proteins (HA, M2 and possibly NA) were detectable on bulged membranes, underneath which RNPs were detected ( Fig. 4a–c , left and middle columns). Slab sections (10-nm thick) revealed that the viral spike proteins were found exclusively at the top of the virion at the initial stage of budding ( Fig. 4d , left column, and Supplementary Fig. S6a ); the rest of the previrion membrane and the plasma membrane proximal to the previrions were smooth, lacking the viral spike proteins. Even at the middle stage of budding, viral spike proteins were restricted to the top to middle portions of the previrions ( Fig. 4d , middle column, and Supplementary Fig. S6b ). The RNPs were suspended from the top of the virion where the viral spike proteins were attached ( Fig. 4d , middle column), suggesting that the viral spike proteins are likely involved in recognition of and association with the RNPs on the plasma membrane as implied by virological studies [21] , [22] . In contrast to previrions in the process of budding, longitudinally sectioned mature progeny virions were almost entirely covered with viral spike proteins ( Fig. 4d , right column, and Supplementary Fig. S6c ). Their RNPs were associated with the interior of the envelope at the top of the mature virion, which is consistent with our previrion findings during the course of budding ( Fig. 4d , left and middle columns). Given that HA, NA or M2 expression alone can form virus-like particles [23] , [24] , [25] , our observations suggest two independent roles for viral spike proteins in virion formation. At the initial stage of virion formation, viral transmembrane proteins (HA, NA and M2) recognize the RNPs. This event is followed by virion shell formation, driven by the viral transmembrane proteins and the M1 protein, which have the intrinsic ability to form the virion shell [25] , [26] , [27] , [28] , leading to the incorporation of the RNPs into virions. 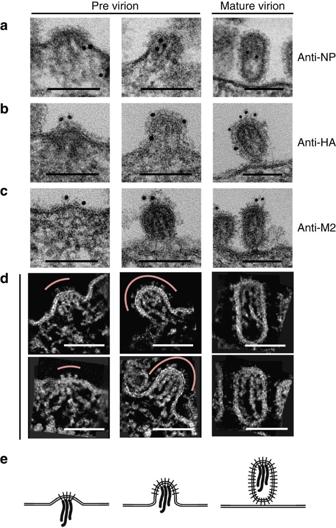Figure 4: Packaging of RNPs into the virion. The left column shows the initial stage of budding, the middle column shows the middle stage and the right column shows mature virions. (a) Immunostaining with an anti-NP antibody conjugated with 10 nm gold beads. (b) Immunostaining with an anti-HA antibody conjugated with 10 nm gold beads. (c) Immunostaining with an anti-M2 antibody conjugated with 10 nm gold beads. (d) Slab slices (10 nm) of previrions in the process of budding and mature virions. Red lines in the left and middle columns indicate the membrane region where viral spike proteins are present. Scale bar, 100 nm. (e) Schematic diagrams of the RNP packaging process. Initial (left), middle (center) and late (right) steps of budding. Figure 4: Packaging of RNPs into the virion. The left column shows the initial stage of budding, the middle column shows the middle stage and the right column shows mature virions. ( a ) Immunostaining with an anti-NP antibody conjugated with 10 nm gold beads. ( b ) Immunostaining with an anti-HA antibody conjugated with 10 nm gold beads. ( c ) Immunostaining with an anti-M2 antibody conjugated with 10 nm gold beads. ( d ) Slab slices (10 nm) of previrions in the process of budding and mature virions. Red lines in the left and middle columns indicate the membrane region where viral spike proteins are present. Scale bar, 100 nm. ( e ) Schematic diagrams of the RNP packaging process. Initial (left), middle (center) and late (right) steps of budding. Full size image The 3-D structure of RNPs within progeny virions provides clues to the mechanisms by which the segmented RNPs are packaged into progeny influenza virions. Here, by using STEM, we constructed and analysed the 3-D structure of 30 progeny virions, all of which possessed the eight RNPs in a well-organized arrangement. This observation strongly suggests that the packaging of a set of eight RNPs generally occurs in each virion, clearly supporting a selective packaging model in which a complete set of eight vRNA segments is selectively packaged into each progeny virion [15] , [16] , [17] . In addition to virological evidence from reverse genetics studies, showing that mutations or deletions in a packaging signal of a vRNA segment reduce incorporation of the other vRNA segments into progeny virions [29] , [30] , [31] , [32] , [33] , [34] , we demonstrated structurally that physical associations occur among the eight RNPs. The associations may reflect specific interactions among vRNA segments to assemble and maintain a distinct structural arrangement of the eight RNPs. Accordingly, the eight RNPs would be assembled in the nucleus or cytoplasm before being packaged into progeny virions, and incorporated into progeny virions as an interlinked complex of eight RNPs, not as eight independent RNPs. Such associations may be at least partially maintained even after progeny virions bud from infected cells, as eight RNPs are sometimes found to be arranged in the '7+1' organization within purified virions [14] , [35] , [36] . Previous studies have reported that deletion of the cytoplasmic tail of HA, NA or M2 leads to a reduction in the amount of NP protein in virus particles [21] , [22] , although it is unclear how the deletion of these spike proteins reduces incorporation of the NP protein into virions. The current EM data suggest that viral spike proteins, such as HA and M2, appear to be involved in the association of the well-ordered eight RNPs at the initial step of budding ( Fig. 4e , left). Because previous virological studies have shown that virions with a complete set of eight RNPs are more efficiently produced than those with less RNPs [15] , [30] , [31] , the well-ordered eight RNPs, rather than individual RNPs, may be preferentially recognized by these spike proteins on plasma membrane and efficiently packaged into progeny virions. In most of the virions reconstructed here, we could not measure the exact lengths of the RNPs within the virions, because the ends of the three long RNPs were often excluded from the 200-nm thick sections and it was technically difficult to distinguish between the RNPs and the M1 protein/lipid envelope at the budding tip of the virions due to their similar electron densities. We therefore measured differences in length between the RNPs to ascertain the accuracy of the size classification of the RNPs. The differences in length between the respective RNP pairs were similar among 30 virions ( Supplementary Fig. S3 ), suggesting that the assignment of the RNPs is reliable. Short defective vRNA segments could potentially compromise this analysis. To eliminate this possibility, we attempted to detect short vRNA by extracting, gel separating and silver staining them in virions produced under the same conditions as the STEM tomography was performed for budding virions ( Supplementary Fig. S7 ). However, we did not detect such vRNAs. Therefore, the assignment of the eight RNPs in this study is reliable. Here, we demonstrated that all 30 virions contained three long RNPs and five shorter RNPs of statistically different lengths, strongly suggesting that all virions contain eight different kinds of vRNAs segments. However, the differences in length between the RNPs were not proportional to the differences in nucleotide length of the vRNA segments ( Supplementary Fig. S3a ). Although the exact reason for this discrepancy is unknown, there may be an important biological reason for this observation; for example, it is possible for specific transverse interactions among the RNPs to distort their rod-like structures, thereby causing longitudinal changes in RNP length. Interestingly, the distinct positioning of the eight RNPs was not consistent among the 30 different virions examined here, although there was a certain pattern for the positions of the four longer RNPs ( Fig. 3 ; Supplementary Fig. S4 ). This finding suggests that the four longer RNPs (probably the PB2, PB1, PA and HA vRNA segments based on their number of nucleotides) have important roles in forming the multi-segment complex and that the interactions between the RNPs are not simply one-on-one, but more complex. Although the exact mechanisms for the specific interactions among the RNPs to form the multi-segment complex remain a mystery, unveiling the packaging mechanisms of the segmented influenza virus genome in detail will provide us with not only fundamental knowledge of general virology but also new strategies to combat seasonal and pandemic influenza. Cells and viruses A stock of A/WSN/33 (H1N1) was prepared by growing the virus in Madin–Darby canine kidney (MDCK) cells. Preparation of thin sections Preparation for chemical-fixed samples was performed as described [8] . For rapid freezing, the virus-infected MDCK cells were rapidly frozen using an EM PACT II (Leica Microsystems, Vienna, Austria) and were freeze-substituted with 1% uranyl acetate in dry acetone at −90 °C in a temperature-controlling device, EM AFS II (Leica Microsystems). After dehydration with a series of ethanol gradients, the samples were processed for conventional EPON embedding. Thin sections (approximately 200 or 100 nm) were stained with 2% uranyl acetate and Reynold's lead and then coated with carbon on both sides. Before imaging, the thin sections were plasma-cleaned (Plasma cleaner model 1020, Fischione, Export, PA, USA). STEM tomography and image analysis The tilt series was recorded with a 200-kV field emission STEM (Tecnai F20, FEI, Eindhoven, the Netherlands) by using an annular dark-field detector (Fischione). The digital images were taken with a 2cos θ ° increment over a ±70 range with a pixel size ranging from 0.25 to 1 nm. Tomograms were reconstructed by using the simultaneous iterative reconstruction technique and Inspect3D software (FEI). For the dual-axis tilt series, the x and y axis tilt series were reconstructed separately as described above and combined by using Inspect3D software (FEI). The volume segmentation, visualization, snap-shot capture, movie creation and slab slice creation were performed with the Avizo 6.2 image processing package (Visualization Science Group, Burlington, MA, USA). Segmentation was performed based on the density and morphological characteristics of the RNPs by using both automatic (the 'magic wand') and manual (the 'brush') tools. Probability calculations for the order of RNPs The probability (P1) that a long RNP is present at the center of the multi-segment complex was calculated as shown below, where a long RNP was categorized as number 3 or 4; ' n ' represents the total number of virions, which was 30 in this study. The probability (P2) that three long RNPs line up sequentially among the seven peripheral RNPs was calculated as shown, given that a long RNP is present at the center of the multi-segment complex. The probability (P3) that the three long RNPs do not line up sequentially among the seven peripheral RNPs was calculated as shown; ' n ' represents the total number of virions, which was 30 in this study. Immuno EM Immuno EM against RNP was performed as described [8] . For immuno EM against the HA and M2 proteins, virus-infected cells were fixed with 4% paraformaldehyde and immunostained with an anti-HA or anti-M2 monoclonal antibody, followed by incubation with 10 nm gold-conjugated goat anti-mouse IgG. After immunostaining, the samples were processed for conventional thin-section EM as described [8] . Thin sections were stained with 2% uranyl acetate and Reynold's lead and examined with a Tecnai F20 transmission EM (FEI) operated at 80 kV. Acrylamide gel electrophoresis MDCK cells were infected with virus at a multiplicity of infection of more than 10 as described previously [8] . Twenty-four hours later, budding virions were purified by ultracentrifugation through 20% (w/w) sucrose and suspended in phosphate-buffered saline. Viral RNA was extracted by using an RNeasy Mini Kit (Qiagen, Hilden, Germany), separated by electrophoresis in a 4% polyacrylamide gel with 7 M urea, and then visualized by using a Clear stain Ag kit (Wako Pure Chemical Industries, Osaka, Japan). How to cite this article: Noda, T. et al . Three-dimensional analysis of ribonucleoprotein complexes in influenza A virus. Nat. Commun. 3:639 doi: 10.1038/ncomms1647 (2012).